Structural basis for recognition of autophagic receptor NDP52 by the sugar receptor galectin-8 Infectious bacteria are cleared from mammalian cells by host autophagy in combination with other upstream cellular components, such as the autophagic receptor NDP52 and sugar receptor galectin-8. However, the detailed molecular basis of the interaction between these two receptors remains to be elucidated. Here, we report the biochemical characterization of both NDP52 and galectin-8 as well as the crystal structure of galectin-8 complexed with an NDP52 peptide. The unexpected observation of nicotinamide adenine dinucleotide located at the carbohydrate-binding site expands our knowledge of the sugar-binding specificity of galectin-8. The NDP52–galectin-8 complex structure explains the key determinants for recognition on both receptors and defines a special orientation of N- and C-terminal carbohydrate recognition domains of galectin-8. Dimeric NDP52 forms a ternary complex with two monomeric galectin-8 molecules as well as two LC3C molecules. These results lay the groundwork for understanding how host cells target bacterial pathogens for autophagy. Autophagy is a bulk degradation process for cellular components that recycles macromolecules and maintains cellular homeostasis [1] , [2] . In contrast to nonspecific and bulk autophagy, selective autophagy involves targeted recognition and removal of various cellular structures, including protein aggregates, various cellular organelles and intracellular pathogens [2] , [3] , [4] . For this selective process, autophagic receptors that simultaneously bind target substrates and the key autophagic molecule Atg8 (LC3 in mammals) are required [3] . Ubiquitination for proteasomal degradation has long been studied as a key process for determining protein fate [5] and recently it was also found to have a key role in autophagy by marking specific targets for autophagy-mediated degradation [3] , [6] . To date, four ubiquitin (Ub)-binding autophagic receptors (NBR1, p62, optineurin and NDP52 (also known as CALCOCO2)) are known to interact with LC3 through the so-called LC3 interaction region motif [3] , [6] . Crosstalk between autophagy and ubiquitination though p62, NDP52 and optineurin is required for autophagy of the bacterial pathogen Salmonella enterica serovar Typhimurium, which is ubiquitinated by as yet unidentified E3 ligases when the bacterium invades the cytosol [7] , [8] , [9] . Although these autophagic receptors recognize LC3 and Ub through a similar mechanism, they are non-redundant and are recruited independently without interference [5] . NDP52 utilizes its C-terminal Ub-binding zinc finger (UBZ) to recognize Ub on the bacterial surface, and the region between the N-terminal SKIP carboxyl homology (SKICH) domain and central coiled–coil (CC) of NDP52 is responsible for the LC3C interaction [10] , [11] . NDP52 has an intriguing feature in that it binds specifically to GAL8, a sugar receptor, in the region located between the CC and UBZ domains of NDP52 ( [12] ). Galectins are a family of animal lectins that share a characteristic affinity for β-galactosides and similar carbohydrate-recognition domains (CRDs) [13] . Fifteen galectins have been reported to date and are classified into three types: (1) proto, (2) chimera and (3) tandem-repeat [13] , [14] . Proto-type galectins (galectin-1, -2, -5, -7, -10, -11, -13, -14 and -15) have one CRD and form a stable non-covalent homodimer; chimera-type galectin (galectin-3 only) has a non-lectin N-terminal domain and C-terminal CRD (C-CRD); and tandem-repeat-type galectins (galectin-4, -6, -8, -9 and -12) have two homologous CRDs (N-CRD and C-CRD) joined by a variable length linker in a single polypeptide chain. The well-characterized function of galectins is their role in cellular communication as secretory proteins that bind carbohydrates on the cell surface, and in recent years, those in the cytosol have attracted a lot of interest as pattern recognition receptors [13] , [15] . They serve as versatile danger receptors for monitoring endosomal and lysosomal integrity. When S. typhimurium infects host cells, galectin-3, -8 and -9 are recruited into Salmonella -containing vesicles and only galectin-8 (GAL8; also known as LGALS8) is responsible for the restriction of bacteria [12] . The N-terminal CRD (N-CRD) and C-CRD of GAL8 provide different carbohydrate-binding specificity [16] . Indeed, GAL8 specifically senses host glycans through its N-CRD domain after Salmonella -containing vesicles rupture and recruits NDP52 through C-CRD [12] . Therefore, these domains have a critical role in mediating the signals from bacterial infection to autophagic clearance. As noted, there are four autophagic receptors (NBR1, p62, optineurin and NDP52) and 15 galectins in mammals. The autophagic receptors share similar domains for interaction with Ub and LC3, although their molecular architecture is dissimilar [6] , and the galectins possess very similar CRDs in sequence as well as in structure [15] , [17] , [18] , [19] , [20] , [21] . Therefore, the specific interaction between NDP52 and GAL8 remains to be elucidated. To address the molecular basis for the recognition of autophagic receptor NDP52 by GAL8, we describe here the biochemical and structural characterization of the GAL8–NDP52 complex. The details of the interaction between NDP52 and C-CRD of GAL8 were revealed and interestingly, a bound NAD molecule was observed in the sugar-binding site of N-CRD of GAL8. These findings provide insight into the molecular mechanism of relaying the signal from a sugar-binding pattern recognition receptor to an autophagic receptor. Biochemical characterization of NDP52 Our initial crystallization attempt with full-length NDP52 failed, and therefore we further characterized the molecule biochemically. A size-exclusion chromatography with multi-angle light scattering (SEC-MALS) experiment showed that NDP52 behaves as a dimer in solution ( Fig. 1a ). The dimer formation only occurred through the central CC domain ( Supplementary Fig. S1a ) and the remaining domains were not involved in dimerization. When we mixed purified NDP52 with GAL8 and/or LC3C, stable binary (NDP52–GAL8) and ternary (NDP52–GAL8–LC3C) complexes formed with a stoichiometry of 2:2 and 2:2:2, respectively, based on the molecular weight (MW; Fig. 1a ; Supplementary Fig. S1b ). Therefore, monomeric LC3C and GAL8 bind to each monomer of NDP52 ( Fig. 1c ). During this characterization, it was found that residues 372–380 of NDP52 are responsible for the interaction with GAL8 ( [12] ). Thus, a fluorescein isothiocyanate (FITC)-labelled peptide (residues 372–385) was synthesized and its dissociation constant ( K D ) to GAL8 was compared with that of full-length NDP52. The K D of NDP52 was ~0.64 μM based on surface plasmon resonance (SPR; Supplementary Fig. S2 ) and that of the peptide was ~0.51 μM based on fluorescence polarization (FP), indicating similar values using two different techniques. Therefore, we used this peptide for further structural analysis, which we called GAL8-binding region of NDP52 (Galbi). This linker-shortened version of GAL8 is known to be protease-resistant and fully active in vivo [22] , and furthermore, our binding affinity assay using FITC-labelled Galbi peptide showed no difference between the linker-shortened version and intact GAL8 ( Supplementary Fig. S3 ). Therefore, it is simply termed GAL8 here. 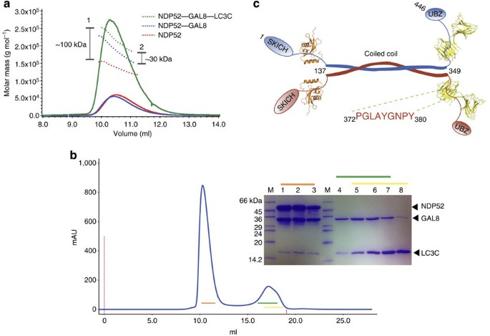Figure 1: A model of the NDP52–GAL8 complex. (a) The ternary NDP52–GAL8–LC3C complex (green line), binary NDP52–GAL8 complex (blue line) and NDP52 complex alone (red line) by SEC-MALS. The dotted line represents measured MW and the vertical bars (1 and 2) indicate the gap in MW. The SEC-MALS result of NDP52 alone (red line) shows that the oligomeric state is ambiguous between dimer and trimer. However, the NDP52–GAL8 complex shows a MW difference of 70 kDa compared with NDP52 alone, which confirmed that two molecules of monomeric GAL8 (MW: ~33.5 kDa;Supplementary Fig. S1b) bound to homodimeric NDP52. Furthermore, the ternary NDP52–GAL8–LC3C complex showed a MW difference of ~30 kDa compared with the binary NDP52–GAL8 complex, which also confirmed that two additional molecules of monomeric LC3C bound to the binary complex. (b) Size-exclusion chromatography data of NDP52–GAL8–LC3C complex. The first peak (marked by an orange bar) represents the ternary complex, as shown by the SDS–polyacrylamide gel electrophoresis (SDS–PAGE) results marked by an orange bar (lane 1, 2 and 3). The second merged peak (marked by green and yellow bar) and corresponding SDS–PAGE results show the remaining free GAL8 (lane 4, 5, 6 and 7) and LC3C (lane 5, 6, 7 and 8). (c) A schematic model of an NDP52 dimer with two LC3Cs (orange) and two GAL8s (yellow). Each monomer is distinguished by red and blue colour, and the ‘PGLAYGNPY’ indicates the amino-acid sequence of the Galbi loop. Figure 1: A model of the NDP52–GAL8 complex. ( a ) The ternary NDP52–GAL8–LC3C complex (green line), binary NDP52–GAL8 complex (blue line) and NDP52 complex alone (red line) by SEC-MALS. The dotted line represents measured MW and the vertical bars (1 and 2) indicate the gap in MW. The SEC-MALS result of NDP52 alone (red line) shows that the oligomeric state is ambiguous between dimer and trimer. However, the NDP52–GAL8 complex shows a MW difference of 70 kDa compared with NDP52 alone, which confirmed that two molecules of monomeric GAL8 (MW: ~33.5 kDa; Supplementary Fig. S1b ) bound to homodimeric NDP52. Furthermore, the ternary NDP52–GAL8–LC3C complex showed a MW difference of ~30 kDa compared with the binary NDP52–GAL8 complex, which also confirmed that two additional molecules of monomeric LC3C bound to the binary complex. ( b ) Size-exclusion chromatography data of NDP52–GAL8–LC3C complex. The first peak (marked by an orange bar) represents the ternary complex, as shown by the SDS–polyacrylamide gel electrophoresis (SDS–PAGE) results marked by an orange bar (lane 1, 2 and 3). The second merged peak (marked by green and yellow bar) and corresponding SDS–PAGE results show the remaining free GAL8 (lane 4, 5, 6 and 7) and LC3C (lane 5, 6, 7 and 8). ( c ) A schematic model of an NDP52 dimer with two LC3Cs (orange) and two GAL8s (yellow). Each monomer is distinguished by red and blue colour, and the ‘PGLAYGNPY’ indicates the amino-acid sequence of the Galbi loop. Full size image Structure of GAL8–Galbi complex The crystal structure of GAL8 identified two separate CRD domains, N-CRD and C-CRD, which share a very similar structure ( Fig. 2a ). Each CRD domain consists of 10–12 β-strands, a 3 10 -helix and connecting loops ( Fig. 2b ). Crystallographically, the GAL8 seemed to form a very unique dimer mediated by the hydrogen bonds forming an antiparallel β-sheet with the first strand β1 from each molecule ( Fig. 2a ). We also analysed the crystalline contacts between N-CRDs for potential dimerization ( Supplementary Fig. S4 ) because it has been reported that GAL8 forms a dimer in vitro through its N-CRD [23] . Furthermore, the proposed dimer models of GAL8 are all different from our observations [19] , [20] . Therefore, we assessed the oligomeric state of GAL8 in solution, which showed clear monomer formation ( Supplementary Fig. S1b ). Interestingly, a portion of the N-terminal segment in N-CRD belongs to C-CRD structurally ( Supplementary Fig. S4 ) and extends to the Galbi peptide-binding region ( Fig. 2a ). The Galbi peptide binds to the C-CRD, which is an opposite side of the carbohydrate-binding site in C-CRD ( Fig. 2b ). Therefore, there is a possibility that only the C-CRD can bind the carbohydrate and peptide simultaneously, but N-CRD is known to be critical for recognizing host glycans after S . Typhimurium infection [12] . Nine residues of the Galbi peptide were all well-defined in the electron density map ( Supplementary Fig. S5a ). The peptide shows a characteristic serpentine shape owing to the high frequency of glycine and proline residues (4/9 residues; Fig. 2c ). In addition, the buried surface area of the GAL8–Galbi complex is ~630 Å 2 . 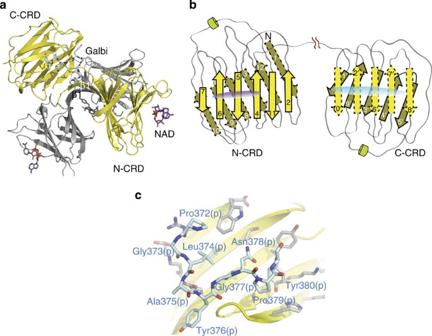Figure 2: Structure of GAL8–Galbi complex. (a) Overall structure of GAL8 with bound Galbi peptide (cyan) and NAD (purple) in the asymmetric unit. The other pair of crystallographic dimer is coloured grey. The first β-strand forming unique interaction is labelled as β1. (b) A topology diagram of GAL8. The β-strands in each N-CRD and C-CRD are numbered sequentially with prime (′) in the C-CRD. The β-strands with a solid line indicate a carbohydrate-binding side in each CRD and those of with a dashed line indicate an opposite side. The elongated purple and cyan ovals indicate NAD- and NDP52-binding sites, respectively. (c) Overall view of Galbi peptide (cyan) bound to the C-CRD of GAL8 (β-strands in yellow and residues in gray). Figure 2: Structure of GAL8–Galbi complex. ( a ) Overall structure of GAL8 with bound Galbi peptide (cyan) and NAD (purple) in the asymmetric unit. The other pair of crystallographic dimer is coloured grey. The first β-strand forming unique interaction is labelled as β1. ( b ) A topology diagram of GAL8. The β-strands in each N-CRD and C-CRD are numbered sequentially with prime (′) in the C-CRD. The β-strands with a solid line indicate a carbohydrate-binding side in each CRD and those of with a dashed line indicate an opposite side. The elongated purple and cyan ovals indicate NAD- and NDP52-binding sites, respectively. ( c ) Overall view of Galbi peptide (cyan) bound to the C-CRD of GAL8 (β-strands in yellow and residues in gray). Full size image Recognition of NDP52 by GAL8 The binding interface between GAL8 and the Galbi peptide is formed largely by hydrophobic residues, including Met1, Val202, Tyr266, Ile270, Tyr272, Lys279, Ala281, Asn283, Gly284 and Trp317 from GAL8 ( Supplementary Table S1 ). A number of polar or charged residues of GAL8 also contribute to the interaction, including Lys204, Glu268 and His286 ( Supplementary Fig. S5b and Supplementary Table S1 ). Residues 372–380 of the Galbi peptide, with the exception of Gly377(p) and Asn378(p), participate in the interaction (‘(p)’ indicates NDP52 residues for clarity). There are also numerous hydrogen bonds involving main chain atoms ( Supplementary Fig. S5b and Supplementary Table S1 ). Three hydrophobic residues, Leu374(p), Tyr376(p) and Tyr380(p), seem to be critically involved in the interaction. Mutation of leucine at position 374(p) to alanine was previously shown to abrogate affinity to GAL8 ( [12] ), and this residue is surrounded by hydrophobic residues Val202, Ile270 and Trp317 from GAL8 ( Fig. 3a ). The side chain of Tyr376(p) extends to the hydrophobic surface of GAL8 formed by side-chain carbon atoms of Asn283 and Tyr266, which is relatively flat ( Supplementary Fig S5a ). Another tyrosine residue, 380(p), seems to be very critical, because it extends into a hydrophobic pocket formed by Tyr272, Lys279 and Ala281 ( Fig. 3b ; Supplementary Fig. S5a ). Furthermore, the hydroxyl group of Tyr380(p) forms a hydrogen bond with the imidazole ring of His286 ( Fig. 3b ). The carbonyl oxygen of Gly373(p) forms a hydrogen bond with the epsilon nitrogen atom of Lys204, and the main-chain nitrogen of Ala375(p) binds with the carboxylic acid of Glu268 ( Fig. 2d ). 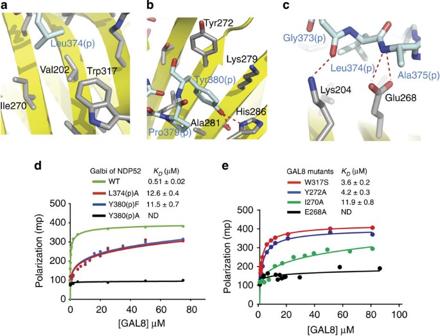Figure 3: Peptide binding and mutagenesis confirming important residues for the interaction. (a) Magnified view showing the detailed interaction around Leu374(p). (b) Magnified view showing the detailed interaction around Tyr380(p). (c) Magnified view showing the importance of main-chain hydrogen bonds of the Galbi peptide. (a–c) Red dashed lines designate hydrogen bonds. (d) An FP assay using FITC-labelled Galbi peptides, including mutants (L374A, Y380F and Y380A) against an increasing concentration of GAL8. (e) An FP assay using a FITC-labelled Galbi peptide against an increasing concentration of GAL8 mutants (E268A, I270A, Y272A and Trp317). (d,e) TheKDvalues were calculated from at least three independent experiments. ND, not determined. Figure 3: Peptide binding and mutagenesis confirming important residues for the interaction. ( a ) Magnified view showing the detailed interaction around Leu374(p). ( b ) Magnified view showing the detailed interaction around Tyr380(p). ( c ) Magnified view showing the importance of main-chain hydrogen bonds of the Galbi peptide. ( a – c ) Red dashed lines designate hydrogen bonds. ( d ) An FP assay using FITC-labelled Galbi peptides, including mutants (L374A, Y380F and Y380A) against an increasing concentration of GAL8. ( e ) An FP assay using a FITC-labelled Galbi peptide against an increasing concentration of GAL8 mutants (E268A, I270A, Y272A and Trp317). ( d , e ) The K D values were calculated from at least three independent experiments. ND, not determined. Full size image Mutagenesis confirms the recognition residues To further dissect this interaction, we generated NDP52 mutants L374(p)A, Y380(p)F and Y380(p)A as well as GAL8 mutants E268A, I270A, Y272A and W317S to assess complex formation. We measured K D values using GAL8- and FITC-labelled mutant Galbi peptides ( Fig. 3d ) as well as GAL8 mutants and wild-type Galbi peptide ( Fig. 3e ). The previously identified mutant L374(p)A had over a 20-fold reduction in binding affinity compared with wild-type (0.51 versus 12.6 μM, respectively; Fig. 3d ). Interestingly, mutation of isoleucine at position 270, which is an interacting residue with Leu374(p), to alanine also showed a similar effect ( Fig. 3e ). Mutation of the C-terminal tryptophan at position 317 to serine based on the sequence alignment between N- and C-CRD ( Fig. 4a ) showed a milder effect as expected because it does not directly interact with Leu374(p). Nevertheless, there was still more than a sevenfold reduction in binding affinity, suggesting that the C-terminal residue of GAL8 has a role in forming a hydrophobic environment ( Fig. 3e ). The Y380(p)F mutant, which removes the hydroxyl group of Tyr380(p), resulted in a similar reduction in affinity (0.51 versus 11.5 μM, respectively), suggesting the importance of this interaction ( Fig. 3d ). The K D values using the SPR technique were very similar (0.64 versus 11.2 μM, respectively; Supplementary Fig. S2 ). The Y380(p)A mutant completely abolished complex formation ( Fig. 3e ), suggesting that it is a critical residue for the GAL8–NDP52 interaction. Mutation of tyrosine at position 272, which is an interacting residue with Y380(p), to alanine showed a milder effect (~8-fold reduction in binding affinity), suggesting that the hydrophobic environment for accommodating the peptide was still maintained partially ( Fig. 3b ). In GAL8, the E268A mutant had no detectable binding affinity, indicating that Glu268 is also a critical residue, especially for interactions with main-chain atoms of NDP52 ( Fig. 3c ). 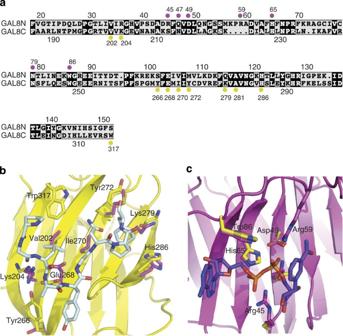Figure 4: Comparison between N-CRD and C-CRD of GAL8. (a) Sequence alignment of N-CRD and C-CRD of GAL8. The residues important for interaction with the Galbi peptide and NAD are marked by yellow and magenta circles, respectively. (b) Detailed view of the peptide-binding site of C-CRD superposed with N-CRD. The residues for the Galbi peptide (cyan) interaction are labelled and the side chains of the corresponding N-CRD residues (magenta) are shown. (c) A detailed view of the NAD-binding site of N-CRD superposed with C-CRD. The residues for NAD (purple) interaction are labelled and the side chains of corresponding C-CRD residues (yellow) are shown. Figure 4: Comparison between N-CRD and C-CRD of GAL8. ( a ) Sequence alignment of N-CRD and C-CRD of GAL8. The residues important for interaction with the Galbi peptide and NAD are marked by yellow and magenta circles, respectively. ( b ) Detailed view of the peptide-binding site of C-CRD superposed with N-CRD. The residues for the Galbi peptide (cyan) interaction are labelled and the side chains of the corresponding N-CRD residues (magenta) are shown. ( c ) A detailed view of the NAD-binding site of N-CRD superposed with C-CRD. The residues for NAD (purple) interaction are labelled and the side chains of corresponding C-CRD residues (yellow) are shown. Full size image Specificity of GAL8 for peptide binding The two CRDs of GAL8 as well as CRDs from other galectins share a high degree of sequence and structural homology ( Fig. 4a ; Supplementary Fig. S6 ) [19] , [20] , [24] . However, our complex structure showed that NDP52 only binds to the C-CRD. Several residues recognizing the Galbi peptide are conserved in the N-CRD and C-CRD (Val202, Glu268 and His286—the same; Lys204, Ile270 and Lys279—similar property), but some differences exist ( Fig. 4a ). The same residues Val202, Glu268 and His286 cannot govern the specificity, and similar residues may not be necessary for peptide-binding specificity. Indeed, our FP experiment using the K204R mutant did not show any binding affinity difference with the wild-type protein ( Supplementary Fig. S7 ). Tyrosine residues 266 and 272 in the C-CRD seem to be critical for Galbi recognition, and the equivalent residues in the N-CRD are Ser102 and Met108, respectively. Both tyrosine residues at these positions are unique in the C-CRD of GAL8 among all galectins ( Supplementary Fig. S6 ). Mutation of tyrosine at position 266 to alanine made the protein unstable and therefore we could not pursue further biochemical analysis. The importance of Tyr272 was confirmed by the K D measurement using the Y272A mutant ( Fig. 3e ). Very interestingly, both terminal residues of GAL8, Met1 and Trp317 are involved in Galbi binding ( Fig. 4b ). As noted, the Met1 N-terminal residue structurally belongs to the C-CRD domain ( Supplementary Fig. S4 ) and the N-terminal region is one of the most variable regions among all galectins ( Supplementary Fig. S6 ). The C-terminal residue of C-CRD in GAL8 is also unique among those of other galectins ( Supplementary Fig. S6 ). The equivalent residue for C-terminal Trp317 in C-CRD of GAL8 is serine in N-CRD of GAL8 and is missing in some galectins ( Supplementary Fig. S6 ). The W317S mutant showed clear reduction in binding affinity ( Fig. 3e ). Indeed, the N- and C-terminus of GAL8 are very close to each other (only 4.4 Å measuring the distance between Cα-atoms) and both are located near the NDP52-binding site ( Supplementary Fig. S4 ). NAD binding of N-CRD The N-CRD of GAL8 is known to preferentially bind to sialylated or sulphated glycans, which is different than all other galectins as well as the C-CRD of GAL8 ( [19] ). Intriguingly, our GAL8 structure showed that an NAD molecule binds to the sugar-binding site of the N-CRD ( Fig. 4c ). The NAD was used as an additive for crystallization and actually had a critical role in crystal packing ( Supplementary Fig. S4 ). However, the clear electron density suggests a specific interaction between N-CRD and NAD ( Supplementary Fig. S8a ). The aromatic ring of Tyr93 in the N-CRD of neighbouring GAL8 in crystal formed a ð-stacking interaction with the adenine ring of NAD, and other protein–protein interactions were observed as well ( Supplementary Fig. S4 ). Therefore, we checked whether dimerization of GAL8 is induced in the presence of NAD. SEC-MALS data of GAL8 and N-CRD of GAL8 in the presence of NAD showed the same result as those in the absence of NAD ( Supplementary Figs S1b and S9 ), suggesting that NAD has no effect on dimerization and also that GAL8 exists as a monomer in solution. The indole ring of Trp86 forms van der Waals contacts with one of the pentose rings of NAD in a similar manner observed in other galectins [13] , [19] , [20] , and the tryptophan residue is strictly conserved among all galectins ( Supplementary Fig. S6 ). The 3′-hydroxyl group of the pentose ring forms a hydrogen bond with the side-chain nitrogen atom of Asn79 ( Supplementary Fig. S8b ). The critical residues for interaction with sulphate or sialic acid moieties of 3′-sialyl and 3′-sulpholactose are positively charged Arg45 and Arg59, respectively, which are responsible for recognizing the negatively charged diphosphate moiety of NAD ( Fig. 4c ). These two arginine residues recognize two phosphate moieties in NAD separately by pairing with Gln47 (for Arg59) and His68 (for Arg45), respectively ( Supplementary Fig. S8b ). Several residues recognizing the sugar binding are conserved in the N-CRD and C-CRD, but these two arginine residues in N-CRD are unique and their equivalent residues in C-CRD are both serine residues ( Supplementary Fig. S6 ). The adenine base and nicotinamide does not participate in the interaction and are exposed to the solvent region. Here, we report biochemical and structural data of the complex between a pattern recognition receptor, GAL8, and an autophagic receptor, NDP52. The NDP52 itself has been known to recognize the Ub-decorated bacteria and invokes autophagic processes [8] , [10] , [25] ; however, mammalian cells possess a system for another line of defense upstream of this process [26] . The ruptured host vesicles expose host glycans, which must be sulphated- or sialylated-galactosides based on the specificity of N-CRD, and this danger signal is then recognized by a very unique lectin, GAL8, among 15 structurally similar galectins. The complexity of this mechanism increases tremendously, because tandem-repeat-type galectins possess two CRDs in a single polypeptide chain. Although no significant structural differences were present within the CRD domains of GAL8 (a root-mean square deviation of 0.3~0.7 Å with 128 matching Cα atoms), superimposition of the C-CRDs only with available GAL8 structures showed dramatic differences in the N-CRD positions, suggesting a diverse spatial arrangement of these two domains ( Fig. 5a ). When we measured the distance among Arg59 residues, which was the major determinant for carbohydrate specificity, this NDP52-bound GAL8 structure showed extreme deviation from other structures ( Fig. 5b ). For example, the N-CRD of our NDP52-bound GAL8 rotates ~49° compared with the GAL8 in complex with lactose in N-CRD (PDB accession code: 4FQZ ), and subsequently a 36.4 Å displacement of the carbohydrate-binding site ( Fig. 5 ). As the first methionine is partially involved in Galbi peptide recognition ( Supplementary Fig. S4 ), we postulate that the special orientation of two separate CRD domains is important for GAL8 function, such as NDP52 binding. We hypothesize that the special orientation of two CRDs for a particular function may be a general feature of tandem-repeat-type galectins. However, further structural studies on other full-length tandem-repeat-type galectins (galectin-4, -6, -9 and -12) are required to confirm this hypothesis. 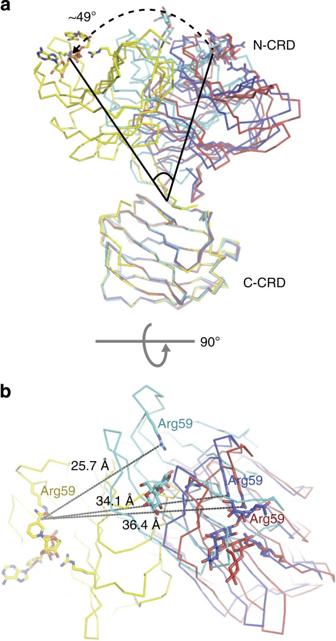Figure 5: Structural comparison among four GAL8 structures. (a) Three GAL8 structures, including both CRDs, are available from PDB (4FQZ—lactose bound in only N-CRD; 3VKL—lactose bound in both N-CRD and C-CRD; 3VKM—sialylated lactose in N-CRD and lactose in C-CRD). The C-CRDs of these Gal8 structures were superposed with that of our Gal8. For clarity, only Cα-traces of each structure (our GAL8—yellow; 4FQZ—red; 3VKM—blue; and 3VKL—cyan) are shown. The large rotation of the N-CRD domain relative to C-CRD compared with the other GAL8 structures is observed in the GAL8–NDP52 complex. A representative angle between N-CRD of our GAL8 and that of the 4FQZ structure is indicated in degrees. (b) A 90° rotation of panel (a) along the horizontal axis showing a top view. Arg59, which is a unique residue of Gal8 N-CRD that provides carbohydrate specificity, is used as a standard for measuring the distance of domain movement. Figure 5: Structural comparison among four GAL8 structures. ( a ) Three GAL8 structures, including both CRDs, are available from PDB (4FQZ—lactose bound in only N-CRD; 3VKL—lactose bound in both N-CRD and C-CRD; 3VKM—sialylated lactose in N-CRD and lactose in C-CRD). The C-CRDs of these Gal8 structures were superposed with that of our Gal8. For clarity, only Cα-traces of each structure (our GAL8—yellow; 4FQZ—red; 3VKM—blue; and 3VKL—cyan) are shown. The large rotation of the N-CRD domain relative to C-CRD compared with the other GAL8 structures is observed in the GAL8–NDP52 complex. A representative angle between N-CRD of our GAL8 and that of the 4FQZ structure is indicated in degrees. ( b ) A 90° rotation of panel ( a ) along the horizontal axis showing a top view. Arg59, which is a unique residue of Gal8 N-CRD that provides carbohydrate specificity, is used as a standard for measuring the distance of domain movement. Full size image The N-terminal Met1 partially interacts with Pro372(p) of NDP52 ( Supplementary Fig. S4 ) and also makes a hydrophobic environment with C-terminal Trp317. It is quite intriguing that both termini of GAL8 cooperatively participate in NDP52 binding by recognizing the N-terminal section of Galbi. As both termini of galectins are diverse in sequence ( Supplementary Fig. S6 ), this must be further investigated. The nine-residue Galbi has a unique three-pronged interaction through hydrophobic residues Leu374(p), Tyr376(p) and Tyr380(p) with GAL8. The key determinant is the C-terminal Tyr380(p) of Galbi based on our structural and biochemical data ( Fig. 3b ). Interestingly, the two tyrosine residues in NDP52, Tyr376(p) and Tyr380(p), specifically interact with two unique tyrosine residues in GAL8, Tyr266 and Tyr272, respectively ( Fig. 4b ). In addition to the hydrophobic interactions described above, the shape complementarity between NDP52 and GAL8 is very characteristic. A similar serpentine shape and the key C-terminal tyrosine residue of the SsrA peptide were found in the structure of the SspB–SsrA complex, although there is no functional linkage between the two protein complexes [27] . Although a charged residue in the middle of the SsrA peptide favors an electrostatic interaction, the hydrophobic Tyr376(p) in Galbi drives the right oriented interaction. Previous in-depth studies of GAL8 showed that its N-CRD is a really unique domain for recognizing sulphated and sialylated sugars [19] , [28] , [29] . In our structure, the diphosphate moiety attached to the pentose ring in NAD binds to the sugar-binding site of N-CRD specifically. There is no apparent functional relevance of the NAD association with the N-CRD of GAL8, but this finding needs further investigation. Indeed, several galectins are recognized as potential targets for both anti-cancer and anti-inflammatory drugs [24] , [30] , [31] , [32] , [33] . As GAL8 is involved in many cellular processes, including cell adhesion, apoptosis, innate immunity and bacterial clearance [12] , [16] , [24] , [34] , it would be useful to develop a small compound to modulate the function of GAL8. Therefore, this NAD-bound GAL8 structure can be used as a template for the design of such a compound. In summary, we have described the detailed molecular characteristics of both NDP52 and GAL8 and show how GAL8 specifically binds to NDP52. Furthermore, the structure of GAL8 has also been described in detail, including NAD binding in the N-CRD. The molecular basis for the interaction between an autophagic receptor and sugar sensor will help us understand how host cells clear invading bacterial pathogens via autophagy in coordination with other host mediators. Note added in proof: The structure of the C-CRD of galectin-8 complexed with an NDP52 peptide has been published very recently [35] . Protein expression and purification Full-length human GAL8 was initially cloned for structural determination. The amplified PCR products treated with restriction enzymes BglII and KpnI were inserted into a modified pET vector for the construction of an N-terminal 6-histidine-tagged protein. The resultant plasmids were transformed into Rosetta(DE3) cells. Protein expression was induced by the addition of 0.5 mM isopropyl-β- D -thiogalactoside at 18 °C for 24 h. Cells were harvested by centrifugation and resuspended in 50 mM HEPES (pH 7.0), 300 mM NaCl and 5 mM imidazole. After sonication, the cell lysate was loaded onto a His-Trap column (GE Healthcare) and then eluted with 30–300 mM imidazole. The histidine tag was cleaved using TEV protease and the resultant proteins (starting with Gly–Ser residues following the first Met) were further purified by ion-exchange column chromatography using 5 ml HiTrap SP FF (GE Healthcare). Finally, proteins were loaded onto a 16/60 Superdex75 gel filtration column (GE Healthcare) pre-equilibrated with 50 mM HEPES (pH 7.0), 200 mM NaCl and 1 mM TCEP. The structural study was not straightforward, and therefore we shortened the long linker between N-CRD (residues Met1–Ser155) and C-CRD (residues Arg184–Trp317) based on previous reports [20] , [22] . This linker-shortened version of GAL8 was overexpressed and purified in a similar manner as the full-length protein. All other proteins, including full-length NDP52, LC3C and NDP52-CC (residues 140–350), were cloned into the modified GST-tagged vector and purified in a similar manner as described above, except that a glutathione-Sepharose 4B affinity column (GE Healthcare) was used instead. Mutant proteins (E268A, I270A, Y272A and Trp317 of GAL8; L374(p)A, Y380(p)F and Y380(p)A of NDP52) were generated using the QuikChange mutagenesis kit (Stratagene), and sample preparation of the mutants was performed in the same way as that of the full-length GAL8 and NDP52. Crystallization and data collection Synthesized Galbi ( 369 RQNPGLAYGNPY 380 ) and FITC-labelled Galbi (FITC-linker- 372 PGLAYGNPYSGIQE 385 ) peptides were purchased from Peptron Inc. Purified GAL8 and Galbi peptides were mixed in a molar ratio of 1:2, respectively, at 4 °C for 30 min and re-loaded onto a gel filtration column to purify the complex. The complex was confirmed by mass spectrometry. Samples were concentrated to 16 mg ml −1 and crystallization was performed by hanging-drop vapour diffusion at 22 °C after mixing an equal volume of reservoir solution containing 0.1 M Tris-HCl (pH 8.5), 30–34% (w/v) PEG400, 200 mM LiSO 4 and 10 mM NAD. Crystals were grown for 2 days and then flash-frozen in liquid nitrogen without any other cryoprotectant. Diffraction data were indexed, integrated and scaled using the HKL2000 software package [36] . Statistics for the collected data are described in Supplementary Table S2 . Structure determination and refinement The GAL8–Galbi complex structure was solved by the molecular replacement method with the program PHASER [37] using the N-CRD of GAL8 as a search model [19] . The molecular replacement solution resulted in four CRD units per asymmetric unit. Initially, the connectivity between these CRD units was not clear. The structure of GAL8 that included N-CRD and C-CRD connectivity was completed by successive cycles of manual rebuilding with COOT [38] followed by refinement using PHENIX [39] . We determined the position of the Galbi peptide using an F o – F c difference Fourier map contoured at 2.0 σ. We built the structure of bound peptide into the electron density map manually, and in this stage, a clear electron density map of NAD at the sugar-binding site of N-CRD was observed. Subsequently, rigid body and restrained refinement were performed with PHENIX [39] . Nine out of 12 residues in the Galbi peptide were built and no electron density was observed for the N-terminal three residues ( Supplementary Fig. S5a ). During the refinement, non-crystallographic symmetry restraints were applied. The assessment of model geometry and assignment of secondary structural elements were achieved using the MolProbity program [40] . Refinement statistics are summarized in Supplementary Table S2 . For interface analysis of the GAL8–Galbi complex structure, the PISA server ( http://www.ebi.ac.uk/msd-srv/prot_int/pistart.html ) and the program LIGPLOT were used [41] , [42] . All figures for the structures were generated using PyMOL ( http://www.pymol.org ). Size-exclusion chromatography with multi-angle light scattering SEC-MALS experiments were performed using a fast protein liquid chromatography system (GE Healthcare) connected to a Wyatt MiniDAWN TREOS MALS instrument and a Wyatt Optilab rEX differential refractometer. A Superdex 200 10/300 GL (GE Healthcare) gel filtration column pre-equilibrated with 20 mM HEPES (pH 7.5), 150 mM NaCl and 1 mM TCEP was normalized using bovine serum albumin protein. Complexed or individual uncomplexed protein, prepared by the methods described earlier, was injected (1–3 mg ml −1 , 0.5 ml) at a flow rate of 0.5 ml min −1 . Data were evaluated using the Zimm model for static light scattering data fitting and represented using an EASI graph with a UV peak in the ASTRA V software (Wyatt). Ternary complex model Based on oligomeric state determination from the SEC-MALS results of the NDP52–GAL8–LC3C complex, a schematic ternary complex model ( Fig. 1c ) was generated as follows. The putative CC region of NDP52 was based on the structure of the ROCK-I CC region (PDB accession code: 3O0Z ) [43] and the structurally uncharacterized SKICH and UBZ domains were shown as ovals. The monomeric forms of LC3C and GAL8 were drawn with the Atg8 structure (PDB accession code: 3RUI ) [44] and this study (PDB accession code: 4HAN ), respectively. FP assay FITC-labelled NDP52 Galbi peptides were dissolved in dimethyl sulphoxide at 2 mM and sequentially diluted with binding buffer (50 mM HEPES (pH 7.0), 200 mM NaCl, 1 mM TCEP and 0.0025% Tween-20) at 5 nM equally in each 100 μl reaction well. Purified GAL8 containing the 6 × His-tag was also serially diluted in binding buffer and mixed into each reaction well at a concentration ranging from 0.5 to 75 μM. Fluorescent measurements to detect the change in light polarization of the FITC-labelled Galbi peptide were performed in a 96-well format on a Molecular Device plate reader with excitation and emission wavelengths of 485 and 530 nm, respectively. A nonlinear graph of GAL8 concentration-dependent polarization was drawn and calculated using GraphPad Prism 6. SPR analysis The molecular interaction between NDP52 and GAL8 was studied using SPR spectrometry (SR7500DC system, Reichert Analytical Instrument). Purified GAL8 was immobilized on a carboxymethyl dextran sensor chip as a ligand. The binding solution of 7.5 μM of either NDP52 WT or Y380F mutant was flowed over the biochip for 3 min (30 μl min −1 ) for molecular association analysis. Subsequently, the washing solution (50 mM HEPES (pH 7.0), 200 mM NaCl and 0.5 mM TCEP) was flowed over the biochip for an additional 3 min (30 μl min −1 ) for molecular dissociation analysis. The association and dissociation rate constants were determined by fitting the binding profiles with the Scrubber 2.0 software provided by the manufacturer. Accession codes: Atomic coordinates and structure factor files have been deposited in the Protein Data Bank under the accession code 4HAN . How to cite this article: Kim, B.-W. et al . Structural basis for recognition of autophagic receptor NDP52 by the sugar receptor GAL8. Nat. Commun. 4:1613 doi: 10.1038/ncomms2606 (2013).